Role of T-cell reconstitution in HIV-1 antiretroviral therapy-induced bone loss HIV infection causes bone loss. We previously reported that immunosuppression-mediated B-cell production of receptor activator of NF-κB ligand (RANKL) coupled with decline in osteoprotegerin correlate with decreased bone mineral density (BMD) in untreated HIV infection. Paradoxically, antiretroviral therapy (ART) worsens bone loss although existing data suggest that such loss is largely independent of specific antiretroviral regimen. This led us to hypothesize that skeletal deterioration following HIV disease reversal with ART may be related to T-cell repopulation and/or immune reconstitution. Here we transplant T cells into immunocompromised mice to mimic ART-induced T-cell expansion. T-cell reconstitution elicits RANKL and TNFα production by B cells and/or T cells, accompanied by enhanced bone resorption and BMD loss. Reconstitution of TNFα- or RANKL-null T-cells and pharmacological TNFα antagonist all protect cortical, but not trabecular bone, revealing complex effects of T-cell reconstitution on bone turnover. These findings suggest T-cell repopulation and/or immune reconstitution as putative mechanisms for bone loss following ART initiation. HIV infection is associated with skeletal deterioration [1] , [2] , [3] , [4] , [5] , [6] . Nearly two-thirds of HIV-infected patients exhibit osteopenia, with osteoporosis occurring in up to 15% of HIV-infected subjects [7] , [8] , [9] . Consequently, an overall —two to fourfold higher prevalence of bone fracture and up to ninefold increase in hip fracture is reported for HIV-infected patients compared with the general population [10] , [11] , [12] , [13] , [14] , [15] . Using an HIV transgenic rat model, we demonstrated that HIV-induced bone loss is related to altered B-cell function [16] presumably via loss of co-stimulation, a consequence of CD4 + T-cell lymphopenia. We recently validated these animal studies in humans, demonstrating a significant increase in B-cell production of the key osteoclastogenic factor, receptor activator of NF-κB ligand (RANKL) and a simultaneous decline in its decoy receptor and physiological antagonist, osteoprotegerin (OPG). The B-cell RANKL/OPG ratio was significantly correlated with bone mineral density (BMD) at the femoral neck and total hip in HIV-infected subjects, suggesting an immunocentric basis for bone loss in HIV infection [17] . Furthermore, studies of T cells in HIV-infected subjects suggest a heightened state of activation that likely further contributes to HIV-induced bone loss [18] . Antiretroviral therapy (ART) causes paradoxical worsening of skeletal health [1] , [2] , [3] , [19] , [20] , [21] . A decline in BMD of up to 6% is observed with ART initiation, a loss comparable to that sustained during the early phase of menopause [19] . Previous attempts to identify the mechanisms of ART-induced bone loss separately from those of HIV itself have been futile, as the direct actions of ART on bone cells in vitro [22] , [23] , [24] and in animal models in vivo [25] frequently fail to recapitulate ART effects observed in HIV-infected patients. Nevertheless, ART drug classes with distinct modes of action mediated through different biochemical pathways are all associated with bone loss [26] , [27] , [28] , suggesting that bone loss is independent of antiretroviral regimen [26] , [29] and implying an indirect effect of ART on bone homeostasis. One such indirect action may be related to HIV disease reversal and homeostatic expansion of the immune cells. In fact, in other non-HIV pathologic conditions such as periodontal disease and postmenopausal osteoporosis, immune activation and inflammation, processes seen during CD4 + T-cell repopulation and expansion with ART, are involved in the pathogenesis of bone loss [30] , [31] , [32] , [33] , [34] . Because of the universality of this bone loss to all ART drug classes, and the known impact of immune activation on bone catabolism in other disease states, an immunocentric explanation for ART-induced bone loss is likely, although has not previously demonstrated. We thus hypothesized that T-cell repopulation and immune reactivation, a consequence of ART-induced HIV disease reversal, may explain the enhanced bone loss following ART initiation. We tested this hypothesis by simulating immune reconstitution in the context of immunodeficiency using T-cell-deficient TCRβ knockout (KO) mice that we reconstituted by adoptive transfer of syngeneic T cells. We show that as with ART-induced T-cell repopulation, a significant increase in bone resorption and a corresponding decline in BMD and cortical and trabecular bone structure follows T-cell reconstitution. Transferred T cells produced significant concentrations of RANKL and TNFα. Furthermore, reconstitution of TNFα- or RANKL-null T cells, as well as treatment with the pharmacological TNFα antagonist Etanercept, led to significant protection of cortical bone, but interestingly, not of trabecular bone. Our data support a role for T-cell reconstitution as a key mechanism of bone loss. We further demonstrated that bone loss associated with disruption of the immuno-skeletal interface could be fully prevented by anti-resorptive medication prophylaxis using zoledronic acid in T-cell-reconstituted animals. Loss of BMD following T-cell reconstitution To investigate whether T-cell repopulation and/or immune reconstitution independently cause bone resorption in the absence of HIV infection or AIDS sequelae, we transplanted CD3 + T cells into genetically identical syngeneic T-cell-deficient TCRβ KO mice by adoptive transfer. T-cell-deficient TCRβ KO mice on a C57BL6 background were injected with vehicle (sham) or reconstituted by adoptive transfer of 1 × 10 5 immunomagnetically purified CD3 + T cells (both CD4 + and CD8 + at physiological ratios). Purified T cells were verified as ⩾ 97% CD3 + by flow cytometry ( Supplementary Fig. 1A ). T-cell number and proliferation were quantitated by flow cytometry 12 weeks later. As expected, T cells had significantly reconstituted in the spleen and bone marrow (BM) after adoptive transfer ( Supplementary Fig. 1B ). Following reconstitution of the TCRβ KO mice, we quantitated BMD using in vivo bone densitometry (dual energy X-ray absorptiometry (DXA)). Over a 12-week period, we observed a dramatic progressive decline in accrual of total body, lumbar spine, femur and tibia BMD in reconstituted mice compared with non-transplanted (sham) TCRβ KO mice ( Fig. 1a–d ), supporting the hypothesis that T-cell repopulation can initiate conditions propitious for bone loss. 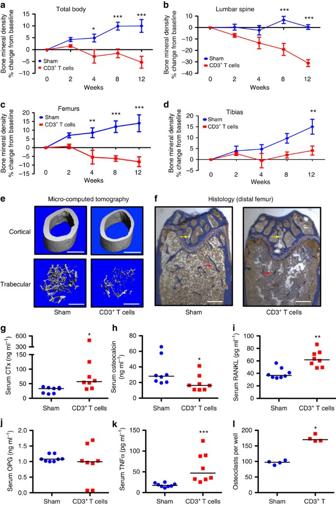Figure 1: T-cell reconstitution induces bone turnover and loss of BMD and bone structure in TCRβ KO mice. BMD (% change from baseline) was quantified by DXA prospectively at baseline, 2, 4, 8 and 12 weeks following T cell (1 × 105CD3+T cells) transplant or vehicle injection (sham) at (a) total body, (b) lumbar spine, (c) femurs and (d) tibias. Data expressed as mean±s.e.m., *P<0.05, **P<0.01, ***P<0.001, two-way analysis of variance with Bonferroni post test (n=8 mice per group). At 12 weeks, the following cross-sectional endpoints were analysed: (e) micro-computed tomography of representative femoral cortical (upper panels) and trabecular (lower panels) high-resolution (6 μm) 3D reconstructions. White bar represents 500 μm. (f) Histological sections of distal femur from sham and CD3+T-cell-reconstituted mice. Mineralized bone stains blue (red arrows indicate trabeculae in the metaphysis and yellow arrows in the epiphysis). White bar represents 200 μm. Serum ELISAs were used to quantify: (g) CTx, (h) osteocalcin, (i) RANKL, (j) OPG and (k) TNFα. Data points represent individual animals with median (black line),n=8 mice per group. *P<0.05, **P<0.01 or ***P<0.001 by Mann–Whitney test. (l)In vitroosteoclastogenesis assay. TRAP+ multinucleated (⩾3 nuclei) cells were generated from bone marrow from four individual mice per group with five wells per mouse averaged per data point. Data representative of two independent experiments and presented as individual wells with median (black line). *P<0.05 by Mann–Whitney test. Figure 1: T-cell reconstitution induces bone turnover and loss of BMD and bone structure in TCRβ KO mice. BMD (% change from baseline) was quantified by DXA prospectively at baseline, 2, 4, 8 and 12 weeks following T cell (1 × 10 5 CD3 + T cells) transplant or vehicle injection (sham) at ( a ) total body, ( b ) lumbar spine, ( c ) femurs and ( d ) tibias. Data expressed as mean±s.e.m., * P <0.05, ** P <0.01, *** P <0.001, two-way analysis of variance with Bonferroni post test ( n =8 mice per group). At 12 weeks, the following cross-sectional endpoints were analysed: ( e ) micro-computed tomography of representative femoral cortical (upper panels) and trabecular (lower panels) high-resolution (6 μm) 3D reconstructions. White bar represents 500 μm. ( f ) Histological sections of distal femur from sham and CD3 + T-cell-reconstituted mice. Mineralized bone stains blue (red arrows indicate trabeculae in the metaphysis and yellow arrows in the epiphysis). White bar represents 200 μm. Serum ELISAs were used to quantify: ( g ) CTx, ( h ) osteocalcin, ( i ) RANKL, ( j ) OPG and ( k ) TNFα. Data points represent individual animals with median (black line), n =8 mice per group. * P <0.05, ** P <0.01 or *** P <0.001 by Mann–Whitney test. ( l ) In vitro osteoclastogenesis assay. TRAP+ multinucleated ( ⩾ 3 nuclei) cells were generated from bone marrow from four individual mice per group with five wells per mouse averaged per data point. Data representative of two independent experiments and presented as individual wells with median (black line). * P <0.05 by Mann–Whitney test. Full size image T-cell induced cortical and trabecular bone loss Trabecular and cortical bone structure were independently quantified in femurs from sham and reconstituted mice 12 weeks after T-cell adoptive transfer, using high-resolution (6 μm) micro-computed tomography (μCT). Representative μCT reconstructions of sham and CD3 + T-cell-reconstituted TCRβ KO femurs ( Fig. 1e ) showed severe deterioration of both trabecular and cortical bone structure. Severely denuded trabecular structure in the femoral epiphysis and metaphysis was also evident on Masson’s Trichrome-stained histological sections ( Fig. 1f ). Quantitative micro-architectural indices of trabecular and cortical structure were further computed from μCT slices ( Table 1 ). Tissue volume (TV), a reflection of bone size, was not significantly altered, however, trabecular bone volume (BV) was drastically reduced in CD3 + T-cell-reconstituted mice, leading to diminished BV fraction (BV/TV), a key index of trabecular bone mass. Trabecular microarchitecture revealed diminished thickness (Tb.Th.) and number (Tb.N. ), and increased trabecular separation (Tb.Sp.) with an overall significant decline in volumetric BMD (TV.D.). T-cell reconstitution was also associated with degradation of cortical bone structure, with significant decline in both cortical area (Ct.Ar.) and thickness (Ct.Th.) two key indices of cortical bone mass. Table 1 Femoral μCT and bone histomorphometry analysis of T-cell-reconstituted mice. Full size table T-cell induced bone turnover, cytokine production and osteoclastogenesis Serum biochemical markers of bone turnover were quantitated in sham- and T-cell-reconstituted TCRβ KO mice 12 weeks after T-cell reconstitution. Bone resorption measured by serum C-terminal telopeptide of type I collagen (CTx) was significantly elevated in T-cell-reconstituted mice ( Fig. 1g ), while bone formation (measured by serum osteocalcin) was modestly, but significantly, suppressed ( Fig. 1h ), consistent with rapid bone loss observed in this model. Serum RANKL, the key osteoclastogenic cytokine ( Fig. 1i ), and its amplifier TNFα ( Fig. 1k ) were significantly elevated in T-cell-reconstituted mice at 12 weeks. Although there was some variability in individual animal responses, overall the RANKL antagonist OPG was not significantly different ( Fig. 1j ) likely leading to an overall increase in the RANKL/OPG ratio, conditions favourable for bone loss. BM from reconstituted mice cultured ex vivo in the absence of exogenous RANKL generated significantly higher numbers of osteoclasts than BM from sham mice ( Fig. 1l ), suggesting a more osteoclastogenic BM microenvironment. Decline in bone formation following T-cell reconstitution To confirm at the tissue level the decline in bone formation following adoptive transfer, we performed quantitative histomorphometry of mouse femurs ( Table 1 ). The number of osteoblasts per bone surface, mineral apposition rate and bone formation rate (BFR/TV) were all significantly diminished. BFR normalized for bone surface (BS) showed a strong negative trend but fell short of statistical significance, likely due to significantly diminished bone surfaces in the transplanted mice. BFR/TV is the index that correlates most closely with bone turnover markers such as osteocalcin [35] . T-cell induced RANKL production To assess whether the increased RANKL observed following T-cell reconstitution was from T cells or other immune cells, we used flow cytometry to evaluate RANKL expression from known major RANKL-producing populations in the spleen and/or BM. We studied T-cell-reconstituted TCRβ KO mice 1 week after T-cell transfer, a time when T cells are undergoing homeostatic expansion and are rapidly repopulating available niches. Representative dot plots of all flow cytometry studies reported below are provided in Supplementary Figs 2–7 . The proportion of CD4 + T cells producing RANKL was significantly elevated in BM ( Fig. 2a ) and spleen ( Fig. 2b ), in reconstituted TCRβ KO mice compared with WT controls. The proportion of BM CD8 + T cells producing RANKL was low in both WT and reconstituted mice ( Fig. 2c ), but the proportion of splenic CD8 + T cells producing RANKL was significantly higher in reconstituted mice ( Fig. 2d ). 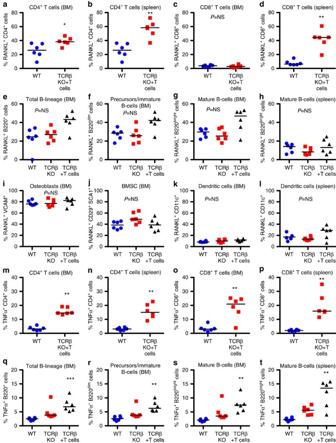Figure 2: Proportion of immune cells producing RANKL and TNFα following T-cell reconstitution. Expression of RANKL was quantified by flow cytometry in WT control mice and TCRβ KO mice 1 week following reconstitution with 1 × 105CD3+T cells (TCRβ+T cells) in: (a) BM CD4+T cells; spleen CD4+T cells; (c) BM CD8+T cells and (d) spleen CD8+T cells. Expression of RANKL was further quantified in: (e) total BM B-lineage; (f) BM immature B cells and B-cell precursors; (g) mature BM B cells; (h) mature B cells in spleen; (i) osteoblasts: (j) BM stromal cells (BMSC); (k) BM dendritic cells and (l) splenic dendritic cells. Expression of TNFα was quantified by flow cytometry in WT control mice and TCRβ KO mice 1 week after reconstitution with T cells (TCRβ+T cells) in: (m) BM CD4+T cells; (n) spleen CD4+T cells; (o) BM CD8+T cells and (p) spleen CD8+T cells. Expression of TNFα was further quantified in: (q) total BM B-lineage; (r) BM immature B cells and B-cell precursors; (s) mature BM B cells; (t) mature B cells in spleen. Data points represent individual animals with median (black line),n=6 independent mice per group. *P<0.05, **P<0.01, ***P<0.001, ****P<0.0001 by Kruskal–Wallis one-way analysis of variance with Dunn's multiple comparison post test for three groups or Mann–Whitney for simple comparisons between two groups. Figure 2: Proportion of immune cells producing RANKL and TNFα following T-cell reconstitution. Expression of RANKL was quantified by flow cytometry in WT control mice and TCRβ KO mice 1 week following reconstitution with 1 × 10 5 CD3 + T cells (TCRβ+T cells) in: ( a ) BM CD4 + T cells; spleen CD4 + T cells; ( c ) BM CD8 + T cells and ( d ) spleen CD8 + T cells. Expression of RANKL was further quantified in: ( e ) total BM B-lineage; ( f ) BM immature B cells and B-cell precursors; ( g ) mature BM B cells; ( h ) mature B cells in spleen; ( i ) osteoblasts: ( j ) BM stromal cells (BMSC); ( k ) BM dendritic cells and ( l ) splenic dendritic cells. Expression of TNFα was quantified by flow cytometry in WT control mice and TCRβ KO mice 1 week after reconstitution with T cells (TCRβ+T cells) in: ( m ) BM CD4 + T cells; ( n ) spleen CD4 + T cells; ( o ) BM CD8 + T cells and ( p ) spleen CD8 + T cells. Expression of TNFα was further quantified in: ( q ) total BM B-lineage; ( r ) BM immature B cells and B-cell precursors; (s) mature BM B cells; ( t ) mature B cells in spleen. Data points represent individual animals with median (black line), n =6 independent mice per group. * P <0.05, ** P <0.01, *** P <0.001, **** P <0.0001 by Kruskal–Wallis one-way analysis of variance with Dunn's multiple comparison post test for three groups or Mann–Whitney for simple comparisons between two groups. Full size image The percentage of total (B220 + ) BM B-lineage cells ( Fig. 2e ), as well as segregated B-cell precursors and immature B cells (B220 dim ) ( Fig. 2f ) and mature B cells (B220 bright ) ( Fig. 2g ) producing RANKL was quantified and although most animals were modestly elevated overall the data fell short of statistical significance. Splenic RANKL production by B cells was lower than for BM overall and no changes or trends were observed in reconstituted mice ( Fig. 2h ). To confirm that the increase in RANKL observed with T-cell reconstitution came from immune cells rather than osteoblasts and their precursors, the BM stromal cells (BMSC), populations long considered to be a rich basal source of RANKL, we assessed the proportion of RANKL-producing osteoblasts (VCAM + cells in the BM) and BMSC (CD29 + SCA1 + cells in the BM) [36] . Approximately 80% of osteoblasts and 40% of BMSC produced RANKL in WT mice but neither population was significantly changed by T-cell reconstitution ( Fig. 2i,j respectively). Dendritic cells were not a significant source of RANKL in WT or reconstituted BM ( Fig. 2k ) or spleen ( Fig. 2l ). B cell and T cell production of TNF We next assessed the cellular sources of elevated TNFα using flow cytometry. The proportion of TNFα-producing BM CD4 + ( Fig. 2m ) and CD8 + ( Fig. 2o ) T cells and splenic CD4 + ( Fig. 2n ) and CD8 + ( Fig. 2p ) T cells were all significantly elevated in reconstituted mice compared with WT. The percentage of total TNFα-producing BM B-lineage cells ( Fig. 2q ), B-cell precursors and immature B cells ( Fig. 2r ), and mature BM ( Fig. 2s ) and splenic ( Fig. 2t ) B cells from T-cell-reconstituted mice was significantly elevated compared with cells from WT mice, but fell short of significance compared with sham-reconstituted TCRβ KO mice. TNFα-producing BM and splenic monocytes/macrophages (CD11b + ) ( Supplementary Fig. 7A,B respectively) were also significantly increased in reconstituted mice relative to WT mice, but despite a strong trend fell short of significance relative to TCRβ KO controls. TNF- or RANKL KO T-cells prevents cortical loss To test the direct contributions of T-cell RANKL and TNFα production to bone loss, we reconstituted 1 × 10 5 CD3 + T cells from either TNFα KO mice or RANKL KO mice into TCRβ KO mice. BMD was quantified at baseline and at 12 weeks after transplant. Reconstitution of TNFα KO or RANKL KO T cells led to partial protection from bone loss compared with WT T cells at total body ( Fig. 3a ), and significant protection of the femurs ( Fig. 3b ) and lumbar spine ( Fig. 3c ). Representative three-dimensional (3D) reconstructions of isolated femurs by μCT ( Fig. 3d ) and quantitative analysis of femoral microarchitecture in Table 2 revealed significant protection from cortical bone loss (both Ct.Ar. and Ct.Th.). RANKL KO T cells showed virtually complete protection, while TNFα KO T cells caused a significantly bunted, bone loss. By contrast, both TNFα and RANKL KO T cells elicited significant trabecular bone loss, with BV/TV indistinguishable from WT T cells and most indices of bone microarchitecture comparable to that of WT T cells. 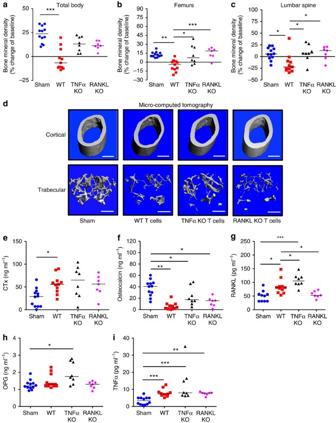Figure 3: Reconstitution of TCRβ KO mice with TNFα KO T cells or RANKL KO T cells blunts cortical but not trabecular bone loss. T-cell adoptive transfer was performed by transplanting 1 × 105WT CD3+T cells, 1 × 105TNFα KO CD3+T cells or 1 × 105RANKL KO CD3+T cells into TCRβ KO mice. BMD was quantified by DXA at baseline and 12 weeks following T-cell transplant at: (a) total body, (b) femurs and (c) lumbar spine. Cross-sectional endpoints were analysed at 12 weeks after transfer for: (d) micro-computed tomography of representative cortical (left panels) and trabecular (right panels) high-resolution (6 μm) 3D reconstructions of femurs. White bar represents 500 μm. Serum ELISAs were used to quantify: (e) CTx, (f) osteocalcin, (g) RANKL, and (h) OPG and (i) TNFα. Data points represent individual animals with median (black line), *P<0.05, **P<0.01, ***P<0.001 by Kruskal–Wallis one-way analysis of variance with Dunn’s multiple comparison post test (n=12 sham, 11 WT, 8 TNFα KO and 7 RANKL KO mice per group). Figure 3: Reconstitution of TCRβ KO mice with TNFα KO T cells or RANKL KO T cells blunts cortical but not trabecular bone loss. T-cell adoptive transfer was performed by transplanting 1 × 10 5 WT CD3 + T cells, 1 × 10 5 TNFα KO CD3 + T cells or 1 × 10 5 RANKL KO CD3 + T cells into TCRβ KO mice. BMD was quantified by DXA at baseline and 12 weeks following T-cell transplant at: ( a ) total body, ( b ) femurs and ( c ) lumbar spine. Cross-sectional endpoints were analysed at 12 weeks after transfer for: ( d ) micro-computed tomography of representative cortical (left panels) and trabecular (right panels) high-resolution (6 μm) 3D reconstructions of femurs. White bar represents 500 μm. Serum ELISAs were used to quantify: ( e ) CTx, ( f ) osteocalcin, ( g ) RANKL, and ( h ) OPG and ( i ) TNFα. Data points represent individual animals with median (black line), * P <0.05, ** P <0.01, *** P <0.001 by Kruskal–Wallis one-way analysis of variance with Dunn’s multiple comparison post test ( n =12 sham, 11 WT, 8 TNFα KO and 7 RANKL KO mice per group). Full size image Table 2 Femoral structural indices in TCRβ KO mice reconstituted with WT, TNFα KO or RANKL KO T cells. Full size table The bone resorption marker CTx ( Fig. 3e ) was significantly increased in the WT T-cell-transplanted group but not in TNFα or RANKL KO groups, although the median values were comparable to that of mice receiving WT T cells, suggesting an overall increased rate of resorption that likely accounts for the trabecular bone loss. Osteocalcin revealed a significant decline in bone formation in WT transplanted T cells and remained significantly depressed in the TNFα and RANKL-null T-cell-transplanted groups ( Fig. 3f ). Serum RANKL ( Fig. 3g ) was increased by transfer of WT T cells and remained elevated in TNFα null T-cell transplant but was not significantly elevated in mice reconstituted with RANKL KO T cells, suggesting that T cells are the major source of RANKL driving bone loss during reconstitution. OPG was not significantly elevated by WT or RANKL KO T-cell transplant but interestingly was significantly increased by transfer of TNFα KO T cells ( Fig. 3h ). As TNFα null T cells did not diminish RANKL concentrations, the data suggest that the mode of action of TNFα in this model is likely to amplify RANKL activity rather than to promote its production. TNFα production ( Fig. 3i ) was significantly increased by WT, TNFα KO and RANKL KO T cells, suggesting that T cells alone do not account for all the TNFα produced, and consistent with our flow analyses. In addition, some mice in this group had unusually high TNFα levels, suggesting that loss of T cell TNFα may promote a compensatory production from other sources. Taken together, these data suggest that production of TNFα and RANKL by T cells contributes significantly to direct cortical bone loss. Interestingly, T-cell production of either TNFα or RANKL was dispensable for trabecular bone loss, possibly due to involvement of other immune cells such as B cells as observed by flow cytometry in Fig. 2 . TNFα ablation blocks cortical but not trabecular, bone loss To assess the significance of global TNFα production in T-cell reconstitution bone loss, mice were treated with the pharmacological TNFα antagonist Etanercept. TCRβ KO mice were injected with vehicle (sham) or reconstituted by adoptive transfer of 1 × 10 5 CD3 + T cells, with or without Etanercept (3 mg kg −1 , three times per week). Prospective BMD quantification over 12 weeks revealed significant bone loss following T-cell reconstitution in the vehicle injected group, but significant protection from bone loss in Etanercept-treated groups at the total body ( Fig. 4a ) and femurs ( Fig. 4c ) with partial protection at tibias ( Fig. 4d ). By contrast, the axial skeleton (lumbar spine), a trabecular-rich site, was not significantly protected by Etanercept ( Fig. 4b ), again suggesting a more pronounced effect of TNFα on cortical than trabecular bone mass. This was verified in the femur by quantifying separate cortical and trabecular microarchitecture by μCT. Representative 3D reconstructions are shown in Fig. 4e with quantitative analysis in Table 3 . As observed for TNFα KO T-cell reconstitution, the TNFα antagonist significantly protected cortical bone thickness and area. Trabecular bone indices including BV/TV revealed partial protection with Etanercept but were not significantly different from either sham or T-cell-reconstituted mice. 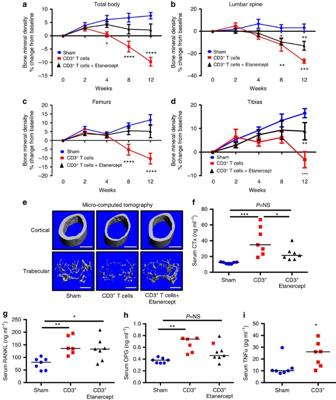Figure 4: Pharmacological TNFα ablation blunts cortical but not trabecular bone loss caused by T-cell reconstitution. TCRβ KO mice were treated with Etanercept, a TNFα decoy receptor, after adoptive transfer of 1 × 105WT CD3+T cells. BMD (% change from baseline) was quantified by DXA prospectively at baseline, 2, 4, 8 and 12 weeks following T-cell (CD3+T cells) transplant or vehicle injection (sham) at (a) total body, (b) lumbar spine, (c) femurs and (d) tibias. Data expressed as mean±s.e.m., *P<0.05, **P<0.01, ***P<0.001, ****P<0.0001 compared with sham by two-way analysis of variance (ANOVA) with Bonferroni post test (n=8 mice per group). Cross-sectional endpoints were analysed at 12 weeks after transplant for: (e) micro-computed tomography. Representative cortical (upper panels) and trabecular (lower panels) high-resolution (6 μm) 3D reconstructions of femurs from T-cell-reconstituted mice, with or without Etanercept at 12 weeks. White bar represents 500 μm. Serum ELISAs were used to quantify: (f) CTx, (h) osteocalcin, (g) RANKL, and (h) OPG and (i) TNFα. Data points represent individual animals with median (black line), *P<0.05, **P<0.01, ***P<0.001 by Kruskal–Wallis one-way ANOVA with Dunn's multiple comparison post test (n=7 mice per group). Figure 4: Pharmacological TNFα ablation blunts cortical but not trabecular bone loss caused by T-cell reconstitution. TCRβ KO mice were treated with Etanercept, a TNFα decoy receptor, after adoptive transfer of 1 × 10 5 WT CD3 + T cells. BMD (% change from baseline) was quantified by DXA prospectively at baseline, 2, 4, 8 and 12 weeks following T-cell (CD3 + T cells) transplant or vehicle injection (sham) at ( a ) total body, ( b ) lumbar spine, ( c ) femurs and ( d ) tibias. Data expressed as mean±s.e.m., * P <0.05, ** P <0.01, *** P <0.001, **** P <0.0001 compared with sham by two-way analysis of variance (ANOVA) with Bonferroni post test ( n =8 mice per group). Cross-sectional endpoints were analysed at 12 weeks after transplant for: ( e ) micro-computed tomography. Representative cortical (upper panels) and trabecular (lower panels) high-resolution (6 μm) 3D reconstructions of femurs from T-cell-reconstituted mice, with or without Etanercept at 12 weeks. White bar represents 500 μm. Serum ELISAs were used to quantify: ( f ) CTx, ( h ) osteocalcin, ( g ) RANKL, and ( h ) OPG and ( i ) TNFα. Data points represent individual animals with median (black line), * P <0.05, ** P <0.01, *** P <0.001 by Kruskal–Wallis one-way ANOVA with Dunn's multiple comparison post test ( n =7 mice per group). Full size image Table 3 Femoral μCT analysis of T-cell-reconstituted mice treated with Etanercept. Full size table Etanercept was further associated with a partial but significant decrease in serum CTx compared with T-cell-reconstituted groups ( Fig. 4f ). By contrast, serum RANKL was not affected by TNFα neutralization ( Fig. 4g ), suggesting that the mode of action of TNFα in this model is likely to amplify RANKL activity rather than promote its production. OPG was also modestly but significantly increased by T-cell transplantation in this experiment and was partially but not significantly reduced by TNFα suppression ( Fig. 4h ). As expected, T-cell adoptive transfer caused a significant increase in TNFα ( Fig. 4i ), however, due to Etanercept cross-reactivity with the enzyme-linked immunosorbent assay (ELISA), we were unable to quantify changes in TNFα production in Etanercept-treated mice. Taken together, these data suggest that TNFα produced by T cells is a significant inducer of cortical bone loss. T-cell number impacts the magnitude of reconstitution bone loss It has been reported that patients with low baseline CD4 count undergo greater bone loss after initiating ART [37] . To determine whether the number of starting T cells affects the extent of bone loss, we adoptively transferred different numbers of CD3 + T cells into TCRβ KO mice and quantified bone turnover and structure after 3 months. Adoptive transfer of a low number (1 × 10 3 ) of T cells produced no significant loss of BMD as quantified by DXA in the lumbar spine ( Fig. 5a ) or femur ( Fig. 5b ), while transfer of a very large number (1 × 10 7 ) produced a small but non-significant loss of BMD in the spine but not femur, compared with 1 × 10 5 T cells that produced significant bone loss at both spine and femur. μCT analysis, however, revealed that high concentrations of T cells produced significant loss of trabecular bone structure, but not of cortical bone (as was reflected by DXA a technique sensitive to cortical but not trabecular bone changes), while the low dose of T cells (1 × 10 3 ) had no significant effect on either compartment ( Fig. 5c and Table 4 ). 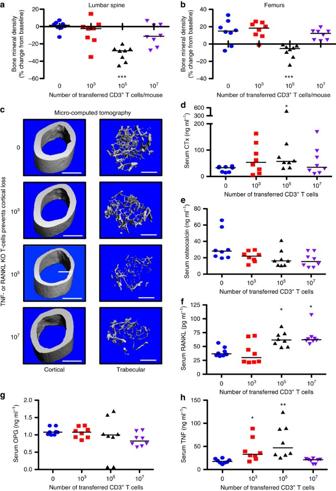Figure 5: Starting T-cell number impacts the magnitude of bone loss in trabecular and cortical bone compartments. T-cell adoptive transfer dose response was performed by transplanting (0, 1 × 103, 1 × 105or 1 × 107) WT CD3+T cells into TCRβ KO mice. BMD was quantified by DXA at baseline and 12 weeks following T-cell transplant at (a) lumbar spine and (b) femurs. Cross-sectional endpoints were analysed at 12 weeks after transplant for: (c) micro-computed tomography or representative cortical (upper panels) and trabecular (lower panels) high-resolution (6 μm) 3D reconstructions of femurs from T-cell-reconstituted mice at 12 weeks. White bar represents 500 μm. Serum ELISAs were used to quantify: (d) CTx, (e) osteocalcin, (f) RANKL, (g) OPG and TNFα (h). Data points represent individual animals with median (black line), *P<0.05, **P<0.01, ***P<0.001 compared with control (0 T cells) by Kruskal–Wallis one-way analysis of variance with Dunn’s multiple comparison post test (n=8 mice per group). Figure 5: Starting T-cell number impacts the magnitude of bone loss in trabecular and cortical bone compartments. T-cell adoptive transfer dose response was performed by transplanting (0, 1 × 10 3 , 1 × 10 5 or 1 × 10 7 ) WT CD3 + T cells into TCRβ KO mice. BMD was quantified by DXA at baseline and 12 weeks following T-cell transplant at ( a ) lumbar spine and ( b ) femurs. Cross-sectional endpoints were analysed at 12 weeks after transplant for: ( c ) micro-computed tomography or representative cortical (upper panels) and trabecular (lower panels) high-resolution (6 μm) 3D reconstructions of femurs from T-cell-reconstituted mice at 12 weeks. White bar represents 500 μm. Serum ELISAs were used to quantify: ( d ) CTx, ( e ) osteocalcin, ( f ) RANKL, ( g ) OPG and TNFα ( h ). Data points represent individual animals with median (black line), * P <0.05, ** P <0.01, *** P <0.001 compared with control (0 T cells) by Kruskal–Wallis one-way analysis of variance with Dunn’s multiple comparison post test ( n =8 mice per group). Full size image Table 4 Femoral structural indices in TCRβ KO mice reconstituted with different numbers of T cells. Full size table Overall, serum CTx was only significantly higher with 1 × 10 5 T cells ( Fig. 5d ) although there was significant variability between individual animals in all transplanted groups. Osteocalcin ( Fig. 5e ) was slightly suppressed relative to sham irrespective of T-cell number although all groups fell short of significance. Serum RANKL ( Fig. 5f ) was significantly increased in both the high (1 × 10 7 ) and moderate (1 × 10 5 ) group, but not the low number of transplanted T cells (1 × 10 3 ). By contrast, serum TNFα concentrations were significantly elevated in moderate (1 × 10 5 ) and low (1 × 10 3 ) groups. Taken together, the data suggest that an increase in RANKL alone is sufficient for trabecular bone loss to occur but TNFα and RANKL are needed for cortical bone loss. This interpretation is consistent with the known action of TNFα on bone, which is to indirectly amplify RANKL-induced osteoclastogenesis and bone resorption, not to promote osteoclastogenesis directly [38] , [39] , [40] . Anti-resorptive therapy reverses T-cell reconstitution bone loss In our final study, we performed a ‘proof-of-concept’ that bone loss associated with T-cell reconstitution can be blocked pharmacologically without impairing T-cell reconstitution. CD3 + T-cell-reconstituted mice were injected once with zoledronic acid (a long-acting anti-resorptive drug approved for amelioration of postmenopausal osteoporosis [41] ) at the time of adoptive transfer and BMD was quantitated by DXA at baseline and at 12 weeks. While T-cell-reconstituted mice lost total body BMD ( Supplementary Fig. 8A ) including at the lumbar spine ( Supplementary Fig. 8B ), femur ( Supplementary Fig. 8C ) and tibia ( Supplementary Fig. 8D ), the zoledronic acid-treated group was protected from bone loss at all sites and actually gained BMD relative to the sham group during follow-up ( Supplementary Fig. 8A–D ). Serum CTx was significantly decreased with zoledronic acid treatment ( Supplementary Fig. 8E ) while osteocalcin remained unchanged ( Supplementary Fig. 8F ). Importantly, at 4 weeks, the proportion of T cells in the peripheral circulation was not significantly different between vehicle and zoledronic acid-treated mice (14.8%±0.2 versus 13.7%±4.0, respectively, N =8 sham and 5 CD3 + T cell per group), suggesting that zoledronic acid does not impede T-cell reconstitution. Although HIV- and ART-induced bone loss has long been recognized, the underlying pathophysiology remains poorly understood. Emerging data suggest that direct HIV effects on the skeleton may be linked to altered immune function including activation of T cells [18] and significant B-cell dysfunction, with consequent increase in the RANKL/OPG ratio, favouring enhanced bone catabolism and loss of BMD [16] , [17] . Immune effects of ART in patients are, however, complex and while some studies suggest that ART may diminish immune activation at least in the short term [42] , [43] , [44] other studies suggest that reversal of inflammation by ART is incomplete and that inflammation persists, albeit at a lower level indefinitely [45] . We now provide a ‘proof-of-concept’ that like HIV infection itself, the bone effect of ART may too have an immunocentric component driving bone loss though a mechanism aligned with immunologic events associated with HIV disease reversal and immune reconstitution and/or reactivation that may lead to persistent low-level chronic inflammation. It is well-established that the immune and skeletal systems are intricately linked via a centralization of common cell types and cytokine mediators—the ‘immuno-skeletal interface’ [16] , [34] , [46] . In HIV-infected patients, suppression of HIV replication with ART leads to a partial recovery of depleted CD4 + T cells through mechanisms involving both peripheral expansion of existing T-cell pools and IL-7-mediated thymic reactivation pathways [47] , [48] . Furthermore, CD4 + T cells are central regulators of adaptive immunity and potently affect the action of other immune cells, including professional antigen-presenting cells (APCs) such as dendritic cells, macrophages and B cells, all of which are capable of secreting TNFα and/or RANKL. In this study, we investigated whether activation of the expanding T-cell pool, together with the reactivation of humoral immunity and antigen presentation to APCs associated with ART-induced disease reversal can lead to constitutive production of key osteoclastogenic cytokines including TNFα and RANKL, tilting the RANKL/OPG ratio in favour of enhanced bone breakdown. To establish a mechanistic basis for immune reconstitution-induced bone loss, we adoptively transferred T cells into an animal model of T-cell immunodeficiency (TCRβ KO mice) to simulate T-cell repopulation, as is likely to occur following ART initiation in HIV-infected patients. We observed a dramatic decline in BMD at all anatomic sites examined following adoptive transfer of a modest number (1 × 10 5 ) of CD3 + T cells supporting the hypothesis that T-cell repopulation can independently induce bone loss in the absence of HIV infection, AIDS pathologies and other confounding risk factors for osteoporosis that coexist in human populations. Consistent with elevated serum RANKL and TNFα, our flow cytometry data suggest that reconstituting T cells are significant sources of RANKL and TNFα. Although CD4 + T cells are severely depleted by HIV infection, significant losses in CD8 + cell populations also occur in advanced HIV infection and recover following ART [49] . To maintain this dynamic, we initially repleted T-cell-deficient mice with both CD8 + and CD4 + T cells in normal physiological ratios (CD3 + ). However, our data revealed that reconstituted CD8 + T cells are also a significant source of RANKL ( Fig. 2d ) and TNFα ( Fig. 2o,p ). As RANKL and TNFα production is associated with T-cell activation, we performed flow cytometry analysis of T cells 3 months after reconstitution and found that the majority of transplanted CD4 + and CD8 + T cells still express the activation marker CD69 and KI-67 a marker of proliferation and synonymous with T-cell activation ( Supplementary Fig. 9 ). These data provide additional support to our hypothesis of long-term bone loss associated with chronic T-cell activation. Furthermore, our data also support a contribution by B cells and monocytes/macrophages, where modest increases were observed. Given the relatively large number of B-cell populations in the BM (25% of nucleated cells) even small increases in RANKL and/or TNFα production may add up to a significant overall contribution to total cytokine levels. Both B cells and macrophages also serve as APCs that normally interact with T cells as part of adaptive immune function. Our data thus suggest that bone loss occurs as a result of a generalized reactivation of the adaptive immune system as a whole following reconstitution of the T cells. This model is outlined diagrammatically in Fig. 6 . 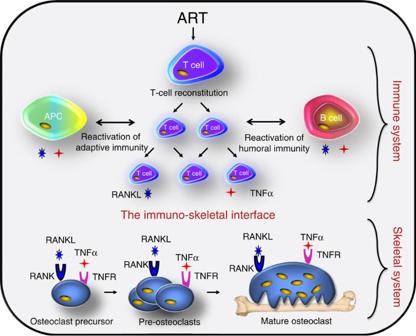Figure 6: Proposed model of ART-induced bone loss. ART-induced T-cell restoration and/or immune reactivation (T-cell/antigen-presenting cell (APC) activity and/or T cell/humoral immunity) leads to osteoclastogenic cytokine production including RANKL and TNFα by T cells and B cells and TNFα by monocytes. These cytokines of immune origin distort the immuno-skeletal interface impacting the skeletal system as RANKL binds to its receptor RANK or osteoclast precursors causing them to differentiate into pre-osteoclasts that fuse into giant multinucleated mature bone-resorbing osteoclasts. The association of TNFα with its receptors on osteoclast lineage cells may further synergize with RANKL signal transduction, thus amplifying osteoclast formation and driving up bone resorption leading to bone loss. Figure 6: Proposed model of ART-induced bone loss. ART-induced T-cell restoration and/or immune reactivation (T-cell/antigen-presenting cell (APC) activity and/or T cell/humoral immunity) leads to osteoclastogenic cytokine production including RANKL and TNFα by T cells and B cells and TNFα by monocytes. These cytokines of immune origin distort the immuno-skeletal interface impacting the skeletal system as RANKL binds to its receptor RANK or osteoclast precursors causing them to differentiate into pre-osteoclasts that fuse into giant multinucleated mature bone-resorbing osteoclasts. The association of TNFα with its receptors on osteoclast lineage cells may further synergize with RANKL signal transduction, thus amplifying osteoclast formation and driving up bone resorption leading to bone loss. Full size image It has been reported that patients with low baseline CD4 count have greater bone loss following ART initiation [37] , suggesting that the extent of homeostatic repopulation may have an impact on bone turnover. Interestingly, the number of T cells reconstituted did indeed have a significant and complex effect on bone loss as a modest number of starting T cells elicited severe bone loss in contrast to very low and very high numbers. Furthermore, very high numbers of T cells induced severe trabecular, but not cortical bone loss, while modest T-cell numbers caused loss in both compartments. Very low numbers of T cells did not induce significant bone loss consistent with a failure to upregulate RANKL production. Interestingly, TNFα production was significantly elevated in this group, but was insufficient to promote bone loss in the absence of increase RANKL. These data are consistent with the action of TNFα, which is not directly osteoclastogenic but functions to synergistically amplify the activity of RANKL [38] , [39] , [40] . Another interesting observation is that very high concentrations of transferred T cells produced RANKL production but not TNFα and led to trabecular, but not cortical, bone loss. The amplificatory role of TNFα thus appears to be essential to amplify RANKL to induce a robust cortical bone loss. Indeed transplantation of T cells deficient in TNFα production likewise led to only trabecular bone loss. These data are further consistent with the fact that pharmacological ablation of TNFα using Etanercept also significantly protected cortical bone, while mediating only weak protection of trabecular bone mass. The transplantation of T cells deficient in RANKL production led to complete protection of cortical bone, however, surprisingly did not provide significant protection from trabecular bone loss. These data suggest that additional sources of RANKL such as those from B cells may be sufficient to promote trabecular bone loss in the presence of permissive concentrations of TNFα. The reason that different concentrations of T cells lead to somewhat different cytokine production and bone loss is not presently clear, however, we speculate that higher doses of T cells may lead to reconstitution too rapidly to generate sufficient prolonged TNFα production, while too few T cells may produce inadequate concentrations of RANKL to effectively drive bone loss. Another plausible explanation is that the expansion of T cells from a modest pool may lead to a contraction of the T-cell repertoire and accumulation of a relatively large number of T-cell clones responding robustly to foreign and self-antigens. Although rare, such reactive T-cell clones would likely have a selective advantage and more effectively reconstitute than non-reactive clones, leading to their preferential amplification. High concentrations of reactive T-cell populations could mediate a persistent inflammatory response. Persistent inflammation is indeed a well-documented feature of patients on long-term ART [45] , [50] , and although the cause is unclear our mouse model may indeed be replicating this event. A similar effect is observed in aging (inflammaging) due to age-associated contraction of the T-cell repertoire leading to accumulation of autoreactive T cells [51] and bone loss. This explanation is consistent with our observations of chronic bone loss persisting for at least 3 months in mice, time points well beyond the 2–3 week time frame normally required for homeostatic expansion to be completed following adoptive transfer. The fact that not only T cells produce RANKL and/or TNFα, but also multiple other immune cells including APCs, B cells and monocytes, suggests that chronic activation of immune responses may underlie long-term bone loss. It is important to point out that bone loss in HIV-infected patients on ART is also polymorphic and that even within a defined cohort there are subjects who are resistant to bone loss and other with extensive bone loss. The factors playing into this are likely complex and multifactorial but the extent of T-cell reconstitution, number of starting and ending T cells, and other immune cells, may well play into the eventual outcome. Eight-week-old mice were used for adoptive transfer, a time at which the long bones are still growing and accreting bone mass. As a consequence, T-cell adoptive transfer leads to a significant delta between sham and experimental groups as a consequence of both bone loss and a failure to accrete new bone mass. These femoral data may provide clues as to the effects of T-cell reconstitution on bone modelling in children initiating ART. However, as vertebral BMD peaks earlier (around 8 to 12 weeks) in this strain, reconstituted animals show a significant loss of BMD that may more closely represent bone remodelling in adult humans initiating ART. The TCRβ KO mouse, however, is a thymus independent model of T-cell deficiency and despite the relatively young age of the mice the T-cell reconstitution phase of the study is likely representative of human adults where the thymus is expected to be largely atrophic and unlikely to significantly contribute to T-cell restoration. Competition from de novo T-cell generation through the thymus may significantly alter the dynamic in children and remains to be studied. Since the majority of HIV-infected adults have declining bone mass due to natural aging, interventions to prevent further bone loss are needed in this population. The transient and early increase in bone resorption following ART-initiation [19] , [52] suggests a potential for short-term anti-resorptive therapy, for which we provide a proof-of-concept in T-cell-reconstituted mice. Importantly, zoledronic acid did not impair T-cell reconstitution in these immunodeficient mice. Therefore, short-term use of this and related bone protective agents may be safe in HIV-infected patients initiating ART. In fact, zoledronic acid has been used successfully in the treatment of osteoporosis in HIV-infected patients [53] , [54] and extending treatment pre-emptively to protect against ART-associated bone loss, even in non-osteoporotic patients, may be an important future approach to reducing fracture in this at risk population. Immune reconstitution in mice led to not only cortical, but also dramatic trabecular bone loss, even under conditions where cortical bone loss was not induced. It is important to note that traditional DXA-based bone densitometry measurements in patients significantly underestimate trabecular bone loss and may thus underestimate the extent of total bone loss and hence fracture risk. This is especially problematic in younger populations where fracture risk does not directly correlate with BMD T -scores [55] , leading to a conservative approach to therapy. Although our animal model may not completely recapitulate the complexity of HIV infection state and the effect of ART in humans, it does offer a unique opportunity to isolate the bone impact of immune reconstitution in a background of immunodeficiency without the plethora of confounding variables that plague clinical studies in human. In conclusion, our data demonstrate a cause-effect relationship between T-cell repopulation and/or immune reconstitution and osteoclastic bone loss. These data provide a proof-of-concept that enhanced bone loss associated with ART initiation may be related, in large part, to immune regeneration and/or reactivation rather than, or in addition to, direct effects of ART on bone cells. In our animal model, short-term anti-resorptive therapy prevented bone loss associated with T-cell repopulation and should be explored further in HIV-infected patients starting ART. Mice All animal studies were approved by the Emory University Institutional Animal Care and Use Committee (IACUC) and were conducted in accordance with the National Institutes of Health Laboratory Guide for the Care and Use of Laboratory Animals. Mice were housed under specific pathogen-free conditions and were fed gamma-irradiated 5V02 mouse chow (Purina Mills) and autoclaved water ad libitum . The animal facility was kept at 23 °C (±1 °C) with 50% relative humidity and a 12:12 h light/dark cycle. Animals were distributed into experimental groups based on baseline BMD measurements of lumbar spine and femurs to minimize variances in total BMD between groups that could bias outcomes in cross-sectional studies such as in vitro μCT and histomorphometry. T-cell adoptive transfer CD3 + T cells were purified from the spleens of 6–8-week-old female WT C57BL6 mice. For some studies, T cells were harvested from 6–8-week-old female TNFα KO C57BL6 mice purchased from Jackson Labs (Bar Harbor, ME) or 6–8-week-old female RANKL KO mice on the C57BL6 background. RANKL KO mice were obtained from an Emory breeding colony derived from donors originally provided by Dr Yongwon Choi (the University of Pennsylvania) [56] , [57] . T cells were purified by negative immunomagnetic isolation (Stem Cell Inc.) to ⩾ 97% purity ( Supplementary Fig. 1A ). All buffers, reagents and materials used in T-cell purification were sterile and endotoxin free, and T cells were processed under sterile conditions. Unless otherwise stated 1 × 10 5 purified T cells were adoptively transferred by tail vein injection into syngeneic female C57BL6 TCRβ KO mice at 8 weeks of age. Sham mice were tail vein injected with vehicle (phosphate-buffered saline (PBS)). Where indicated, mice received a single 0.4 mg kg −1 i.p. dose of zoledronic acid (Novartis Pharmaceutical Corporation) at the time of T-cell adoptive transfer. Some T-cell-reconstituted TCRβ KO mice were injected i.p. 3 times per week for 3 months with 3 mg kg −1 of the pharmacological TNFα antagonist Etanercept (Pfizer Inc.). Mice were killed 3 months after adoptive transfer for detailed bone and immuno-phenotyping. Bone densitometry BMD measurements were performed in anesthetized mice at baseline (0) and at 2, 4, 8 and 12 weeks following sham or T-cell reconstitution by DXA using a PIXImus 2 bone densitometer (GE Medical Systems) as described [58] . Data are presented as percentage change from baseline for each mouse. Baseline BMD (g cm −2 ) for each mouse in each group are located in Supplementary Tables 1–4 . Micro-computed tomography μCT was performed in femurs ex vivo using a μCT40 scanner that was calibrated weekly with a factory-supplied phantom (Scanco Medical, Bassersdorf, Switzerland) as described [58] , [59] . For trabecular bone, 100 tomographic slices were taken (total area of 600 μm) at the distal right femoral metaphysis at a voxel size of 6 μm (70 kVp and 114 mA, and 200 ms integration time). Trabecular bone was segmented from the cortical shell, for a total area of 0.6 mm beginning ∼ 0.5 mm from the distal growth plate and projection images reconstructed using the autocontour function for trabecular bone. Cortical bone was quantified at the mid-diathesis from 100 slices at a voxel size of 6 μm. Representative samples were reconstructed in 3D to generate visual representations of cortical and trabecular structure. Indices and units are standardized per the ‘Guidelines for assessment of bone microstructure in rodents using μCT’ [60] . Quantitative bone histomorphometry Bone histomorphometric analysis was performed at the University of Alabama at Birmingham Center for Metabolic Bone Disease-Histomorphometry and Molecular Analysis Core Laboratory, as previously described by us [59] , [61] . Briefly trichrome-stained plastic-embedded sections of calcein double labelled femora from sham and CD3 + T-cell-reconstituted mice were analysed by an operator blinded as to the nature of the samples. Indices and units are reported per the revised recommendations of the ASBMR Histomorphometry Nomenclature Committee [62] . Biochemical indices of bone resorption CTx, Osteocalcin, total RANKL, OPG and TNFα were quantified in mice serum 12 weeks after T-cell transfer using RATlaps (CTx) and Rat-MID (osteocalcin) ELISAs (Immunodiagnostic Systems Inc. Fountain Hills AZ) and ELISAs from R&D Systems for RANKL, OPG and TNFα. In vitro osteoclastogenesis assays Whole BM was cultured in αMEM supplemented with 10% foetal bovine serum (FBS) and treated with rmM-CSF (30 μg ml −1 ). After 9 days, TRAP + multinucleated cells ( ⩾ 3 nuclei) were quantitated under light microscopy and normalized for size based on number of nuclei. Flow cytometry Surface staining . Single cell suspensions of spleens and BM were prepared and surface staining was performed on 1 × 10 6 cells per reaction in FACS buffer (PBS containing 1% FBS) for 30 min at 4 °C followed by one wash in FACS buffer and fixation in PBS containing 1% paraformaldehyde. All antibodies were purchased from eBioscience Inc. (San Diego, CA), unless otherwise indicated. For direct staining of T cells, we used rat anti-mouse CD4-FITC (clone Gk1.5, 0.25 μg per test) and CD8-APC (clone 53-6.7, 0.125 μg per test); B cells were stained using cd45R (B220)-FITC (clone RA3–6B2, 0.5 μg per test); monocytes/macrophages were stained using CD11b-APC (cloneM1/70, 0.125 μg per test) and CD11c-APC (clone N418, 0.25 μg per test); myeloid lineage and BMSCs were stained using rat anti-mouse CD106 (VCAM-1)-FITC (clone 429, 0.5 μg per test), Armenian hamster anti-mouse/rat CD29-APC (clone HMb1-1, 0.25 μg per test) and rat anti-mouse Ly-6A/E (Sca-1)-FITC (clone D7, 0.5 μg per test). Rat isotype and fluorochrome-matched controls, as well as fluorescence-minus-one controls were used to control for non-specific binding and to set gates (see Supplementary Figs 10 and 11 ). Indirect surface staining for RANKL was performed as previously described [33] . Briefly, cells were incubated with human OPG-Fc (R&D Systems) at 1 μg ml −1 for 30 min in FACS buffer, followed by anti-human IgG-Fc-PE at 1 μg per test. To ensure specific detection of RANKL, we included controls stained with anti-human IgG Fc-PE without prior pre-incubation with OPG-Fc, and consistently observed negligible background staining levels <5% non-specific binding. Intracellular staining for TNFα production . Cells were cultured unstimulated for 4 h with the protein transport inhibitor Golgistop (BD Biosciences) in 12-well flat-bottomed plates (Costar, Cambridge, MA) at a concentration of 2.5 × 10 6 cells per well in a volume of 2 ml complete medium. The cells were harvested, washed once in FACS buffer and surface stained for lineage markers in FACS buffer as indicated above. After washing the unbound antibody, cells were fixed and permeabilized using the Cytofix/Cytoperm kit according to the manufacturer’s instructions (BD Biosciences). Spontaneous intracellular TNFα production was quantified by flow cytometry using PE-conjugated monoclonal rat anti-mouse TNFα antibody (clone MP6-XT22, 0.125 μg per test). Isotype control antibody (PE rat IgG1, 0.125 μg per test) (BD Biosciences) was used to control for non-specific binding and as a reference to set gates. The minimal number of events for BM CD4 or CD8 subset analysis was 1,250–2,500 cells. Samples were acquired on an Accuri flow cytometer (BD Immunocytometry Systems) and the data analysed with Flowjo software version 9.5.3 (Treestar Inc. Ashland, OR). Statistical analysis Statistical significance was determined using GraphPad Prism 5.0 for Mac (GraphPad Software Inc. La Jolla, CA). Multiple cross-sectional comparisons were performed by Kruskal–Wallis one-way analysis of variance with Dunn’s multiple comparison post hoc test. For simple comparisons between two groups we used the Mann–Whitney test for non-parametric data. Prospective changes over time between two groups were analysed by two-way analysis of variance with Bonferroni post test. P <0.05 was considered statistically significant. How to cite this article: Ofotokun, I. et al . Role of T-cell reconstitution in HIV-1 antiretroviral therapy-induced bone loss. Nat. Commun. 6:8282 doi: 10.1038/ncomms9282 (2015).